A unified design space of synthetic stripe-forming networks Synthetic biology is a promising tool to study the function and properties of gene regulatory networks. Gene circuits with predefined behaviours have been successfully built and modelled, but largely on a case-by-case basis. Here we go beyond individual networks and explore both computationally and synthetically the design space of possible dynamical mechanisms for 3-node stripe-forming networks. First, we computationally test every possible 3-node network for stripe formation in a morphogen gradient. We discover four different dynamical mechanisms to form a stripe and identify the minimal network of each group. Next, with the help of newly established engineering criteria we build these four networks synthetically and show that they indeed operate with four fundamentally distinct mechanisms. Finally, this close match between theory and experiment allows us to infer and subsequently build a 2-node network that represents the archetype of the explored design space. Synthetic biology aims at engineering tunable gene circuits, with standardized components [1] , [2] , [3] , [4] , [5] , [6] , whose properties then can be extensively studied by combining experiments and computational modelling. Experience gained in this way deepens our understanding of natural networks [7] , [8] , [9] , [10] and widens our perspective on building more complex networks for applications [11] , [12] , [13] , [14] , [15] , [16] , [17] , [18] , [19] , [20] . An important approach in synthetic biology is to screen through many alternative network designs, computationally or experimentally, to find a network capable of achieving a predefined function. However, little attention has been paid to the question of dynamical mechanism. In other words, two successful networks with apparently different regulatory designs may in fact be minor variations of each other from a dynamical perspective—only showing quantitative differences in dynamics. By contrast, two networks with relatively similar designs may operate using qualitatively distinct dynamics. We call these different ways to achieve the same result dynamical mechanisms [21] , as opposed to simply having different network designs (the ‘wiring diagram’ or topology of the network). In general, although there may be many hundreds of different network designs for a given function, there tend to be just a handful of qualitatively distinct dynamical mechanisms, where changing the parameters, rate laws and so on cannot transform one mechanism into another. To explore the broadest range of design options for synthetic biology, it will be important to consider all the qualitatively different dynamical mechanisms, rather than just screening through many different network topologies. We previously developed a computational approach to map dynamical mechanisms for small 3-node networks, performing a predefined regulatory task [21] , [22] . A genotype–phenotype map of this type is far from trivial, due to the non-linear regulatory interactions and feedback loops [23] within the networks. Our goal was to map out the complete list of possible dynamical mechanisms for a given function. The choice of task was inspired by the field of multicellular patterning, in which a gene circuit must interpret a morphogen concentration gradient to make a central spatial stripe [24] , similar to the classic 'French Flag' problem [25] . Only intermediate concentrations of morphogen (and not high or low levels) must activate a target gene, resulting in stripe-forming systems in two dimension. The question of how gene regulatory networks can achieve concentration-dependent responses in a morphogen gradient is a pivotal one in developmental biology and several different mechanisms have been suggested [24] . Isolated networks achieving this function have been built previously [26] , [27] , [28] , [29] , [30] , [31] , [32] , [33] , [34] , but never with the explicit intention of covering and comparing all possible dynamical mechanisms. Our previous theoretical analysis found that this specific task could indeed be performed by multiple different mechanisms [21] . However, key open questions remained: What are the simplest—and yet distinct—dynamical mechanisms or design classes capable of stripe formation? Can we validate them experimentally, even though some of these network mechanisms have not yet been discovered in stripe formation in nature? By taking this broad design space approach, can we go beyond the case-by-case methodology of synthetic biology, and build instead the complete family of dynamical mechanisms? Can we thus identify individual synthetic components that behave in the same way across different networks, that is, can we identify their universal parameters? Here we follow a three-step approach (theoretical; experimental; modelling) for the effective exploration and creation of successful synthetic circuits. Step 1 is theoretical and involves building a genotype–phenotype map for networks that can produce the desired behaviour. It is important to note that this map is not simply a theoretical screen for identifying all successful topologies, but allows us to distil the handful of qualitatively distinct design classes, which represent all possible dynamical mechanisms for the desired phenotype. Step 2 is to build synthetically these minimal networks for each mechanism, using bacteria. This task requires development of a molecular scaffold to enable the efficient construction of multiple different network designs, and also an extensive set of experimental tests to ensure that the stripe pattern is formed by the dynamical mechanism predicted by the theoretical model. Step 3 is to fit the results of these synthetic networks to a mathematical model and thus closely verify that the distinct dynamics of the theoretical mechanisms are successfully recapitulated in the synthetic circuits. For this purpose, we have developed a quantitative experimental method to track the expression of all three nodes in detail. In addition, we derive mutant networks with altered strengths of regulatory interactions to further confirm the mechanistic basis of each network (16 different circuits are engineered, quantified and modelled for 4 network classes). The success of this procedure allows us to go one step further to find a deeper design principle of stripe formation. Although the dynamics of each design class are different, they all share a common topological feature: they are all incoherent feedforward loop motifs (I-FFLs [35] ), which contain both an activating and a repressing pathway between the morphogen sensor and the stripe gene. We can therefore explore whether a simpler 2-node network—where the stripe gene is directly controlled by both activation and repression from the morphogen sensor gene—replicates this stripe-forming ability in its simplest form. We are successful in building this archetype of I-FFL stripe-forming networks and ultimately discover that it can even display an ‘anti-stripe’ phenotype. Exploring the design space for stripe-forming networks Step 1 of our procedure was theoretical. We created a genotype–phenotype map of stripe-forming networks, by exhaustively enumerating all possible 3-node designs excluding negative autoregulation (2,897 in total). Every network was numerically simulated with 100,000 random parameter sets in a 1D row of virtual cells, using a Hill-like function model of gene regulation based on equilibrium binding of transcription factors to their sites on the promoter [36] ( Supplementary Fig. 1 ). Criteria were defined to select those designs that could create a stripe of expression in the centre of the morphogen gradient (see Supplementary Methods for details). We found that 109 of the possible networks generated a stripe with appropriate parameter values. However, networks with different topologies may in fact operate using the same underlying dynamics. To elucidate this question and aid understanding of how many mechanisms may be present within these 109 designs, we organized them into a complexity atlas [21] ( Fig. 1a , Supplementary Fig. 2 ). In this atlas, each node represents one of the 109 stripe-forming networks and two nodes are connected with a line when they differ by a single interaction (that is, adding or removing one repression or activation). The atlas is thus a ‘metagraph’—a graph of graphs (networks). The nodes of the atlas are laid out such that topological complexity increases upwards, revealing a structure in which four main groups (‘stalactites’) appear. Each stalactite converges downwards to a single network with minimal complexity. Strikingly, these networks correspond to the four known types of incoherent feedforward loops [35] (I-FFL: I1-I4). We explored the temporal dynamics of each minimal mechanism and found them to be distinct in each case (for example, the I1 stripe gene is initially highest on the right-hand side of the field of cells and its peak then shifts to the centre, while in I2 the stripe develops from the centre; Fig. 1b ). Furthermore, phase portraits of these systems and the temporal trajectories also confirm that the four networks achieve the stripe with different dynamical mechanisms ( Fig. 1c ). 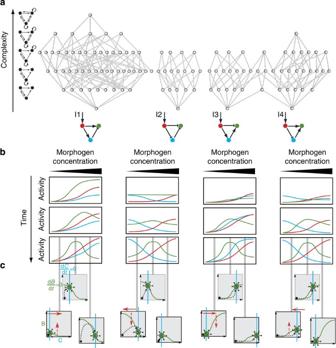Figure 1: Design space of stripe-forming networks. (a) Complexity atlas: grey circles are gene regulatory networks (GRNs) and edges link those with a single connectivity change. The GRNs are laid out such that complexity increases upwards. Examples of networks with the corresponding number of interactions (complexity) are depicted on the left. The bottoms of the ‘stalactites’ represent minimal networks: the four incoherent feedforward loops (I1-I4). Key: arrow, activation; bar, repression; red, morphogen input receiver gene; blue, intermediate loop gene; green, stripe output gene. (b) The temporal development of the three genes were calculated from representative parameters sets of the complexity atlas and shown schematically for each distinct mechanism. (c) Qualitative phase portraits for each distinct mechanism at low, medium and high morphogen concentration. Thexaxis represents the activity of the blue gene (that is, C) and theyaxis, the activity of the green gene (that is, B). The nullcline curves for the blue and green genes (where one variable does not change in time) are shown as coloured lines, and the stable steady state (S) occurs where they intersect (that is, where neither variable changes over time). The black star indicates the initial condition close to the origin. The full red arrows in these phase plots show the nullcline movements in response to the morphogen gradient and the dashed red arrows indicate the increase or decrease in the height of the nullcline. The calculated temporal trajectories are shown as dashed lines, showing why in some cases a low final level for the green gene is preceded by a temporary rise in levels, while in other cases it is not. It is clear from this analysis that mechanisms cannot be smoothly transformed from one into the other, further highlighting the qualitatively different dynamics for each stalactite. Figure 1: Design space of stripe-forming networks. ( a ) Complexity atlas: grey circles are gene regulatory networks (GRNs) and edges link those with a single connectivity change. The GRNs are laid out such that complexity increases upwards. Examples of networks with the corresponding number of interactions (complexity) are depicted on the left. The bottoms of the ‘stalactites’ represent minimal networks: the four incoherent feedforward loops (I1-I4). Key: arrow, activation; bar, repression; red, morphogen input receiver gene; blue, intermediate loop gene; green, stripe output gene. ( b ) The temporal development of the three genes were calculated from representative parameters sets of the complexity atlas and shown schematically for each distinct mechanism. ( c ) Qualitative phase portraits for each distinct mechanism at low, medium and high morphogen concentration. The x axis represents the activity of the blue gene (that is, C) and the y axis, the activity of the green gene (that is, B). The nullcline curves for the blue and green genes (where one variable does not change in time) are shown as coloured lines, and the stable steady state (S) occurs where they intersect (that is, where neither variable changes over time). The black star indicates the initial condition close to the origin. The full red arrows in these phase plots show the nullcline movements in response to the morphogen gradient and the dashed red arrows indicate the increase or decrease in the height of the nullcline. The calculated temporal trajectories are shown as dashed lines, showing why in some cases a low final level for the green gene is preceded by a temporary rise in levels, while in other cases it is not. It is clear from this analysis that mechanisms cannot be smoothly transformed from one into the other, further highlighting the qualitatively different dynamics for each stalactite. Full size image Network scaffold and engineering criteria checklist For Step 2, we built the minimal network of each design class synthetically. A main challenge we faced was to develop a method where components could be consistently reused in different contexts, allowing the exploration of network variants [37] and ideally the full design space. Before building the four networks as synthetic transcription circuits, we therefore designed a general network scaffold strategy for Escherichia coli , consisting of three compatible plasmids ( Fig. 2 ). Each plasmid codes for one node and contains the same multiple cloning sites, for the combinatorial insertion [38] , [39] of promoters, repressor binding sites (operators), ribosomal binding sites, repressors and activators. The arabinose-responsive promoter P BAD receives the input signal (arabinose), whereas superfolder green fluorescent protein (GFP) [40] is the network output, which should form the stripe. T7 and SP6 phage RNA polymerases function as activators from T7 or SP6 promoters [41] , while split T7 RNA polymerase [42] integrates two activations to give an AND gate output (in I4). Negative interactions employ the transcriptional repressors lacI (lactose operon repressor protein) and TetR (tetracycline repressor), placing their operator sites (lacO, TetO) behind promoters. 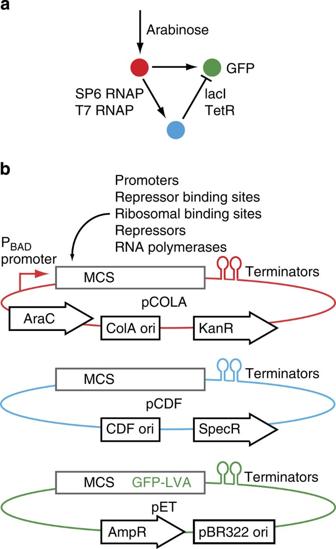Figure 2: Network scaffold. (a) An arabinose-dependent promoter links the concentration-gradient input to a network of activators (T7 and SP6 RNAP) and repressors (lacI and TetR). (b) Each node is encoded on a differentE. coliplasmid (color-coded). Each plasmid contains the same multiple cloning sites (MCS) for the combinatorial insertion of the network components. The plasmids contain compatible origins of replication (ori) and antibiotic resistance cassettes (kanamycin, spectinomycin and ampicillin resistance). The 3-node, 3-plasmid scaffold is described fully inSupplementary Methods. Figure 2: Network scaffold. ( a ) An arabinose-dependent promoter links the concentration-gradient input to a network of activators (T7 and SP6 RNAP) and repressors (lacI and TetR). ( b ) Each node is encoded on a different E. coli plasmid (color-coded). Each plasmid contains the same multiple cloning sites (MCS) for the combinatorial insertion of the network components. The plasmids contain compatible origins of replication (ori) and antibiotic resistance cassettes (kanamycin, spectinomycin and ampicillin resistance). The 3-node, 3-plasmid scaffold is described fully in Supplementary Methods . Full size image While testing the individual components, we observed that strong bacterial stress responses can be induced by expressing synthetic networks at high levels. This metabolic load [43] , [44] can retard growth or decrease global transcription and translation, interfering with synthetic network function. Importantly, a high inducer concentration can even shut down gene expression due to stress, giving an apparent stripe of expression ( Supplementary Fig. 3 ). In other studies, metabolic load has been used reproducibly as a desired property [8] , [45] . However, as our goal was to build four different networks, each functioning with a distinct predefined mechanism, it was essential to exclude metabolic load in each case. Stripes formed due to metabolic load can neither reproduce the appropriate dynamics nor could the model predict the behaviour of mutants. It was therefore critically important to reduce bacterial metabolic burden by using degradation tags and low-activity promoter mutants. We ultimately developed a list of controls or engineering criteria to ensure that our stripes are not caused by metabolic load ( Fig. 3a ). This checklist ensures that networks and mutants behave as predicted. 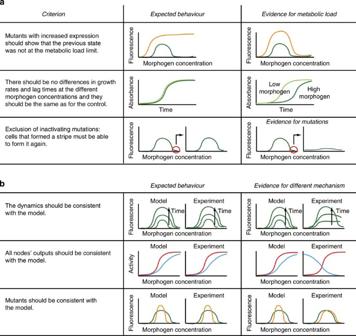Figure 3: Controls for synthetic stripe-forming circuits inE. coli. (a) A list of controls or engineering criteria to verify that an observed stripe is not caused by a bacterial stress response to high network expression (metabolic load;Supplementary Fig. 3). (b) A list of controls to verify the mechanism. Green, wild-type network; orange, mutant network; red, morphogen input receiver gene; blue, intermediate loop gene. Figure 3: Controls for synthetic stripe-forming circuits in E. coli . ( a ) A list of controls or engineering criteria to verify that an observed stripe is not caused by a bacterial stress response to high network expression (metabolic load; Supplementary Fig. 3 ). ( b ) A list of controls to verify the mechanism. Green, wild-type network; orange, mutant network; red, morphogen input receiver gene; blue, intermediate loop gene. Full size image A family of four stripe-forming networks We used our network scaffold to build the minimal stripe-forming I1, I2, I3 and I4 networks synthetically ( Fig. 4 ). The modelling from step 1 not only provided us with the topologies, but also gave us an indication of the relative strengths of the interactions. For example, in I3, we knew the activator between the red and blue nodes had to be weaker than the activator between the blue and green nodes. This knowledge guided our component choices and reduced ‘trial and error’ considerably. We tuned the parameters by using different promoter strengths and repressor binding sites, as well as partially de-repressing lacI and TetR with isopropyl-β- D -thiogalactopyranoside (IPTG) and anhydrotetracycline (aTc), respectively. Screening of circuits was performed on multiwell plates, with each well containing a different concentration of arabinose, and monitoring GFP levels over time gave stripe gene readouts. All networks passed the metabolic load control checklist of Fig. 3a ( Supplementary Figs 4–6 ). In addition, the temporal dynamics of formation of the stripe were measured ( Fig. 4d ) and showed good qualitative agreement with the predictions ( Fig. 1 ). To confirm that each network was capable of true spatial patterning, we also placed a localized source of arabinose on a two-dimensional bacterial lawn, and observed a discrete ring of GFP fluorescence at a fixed distance from the source [28] , [31] ( Fig. 4c ). 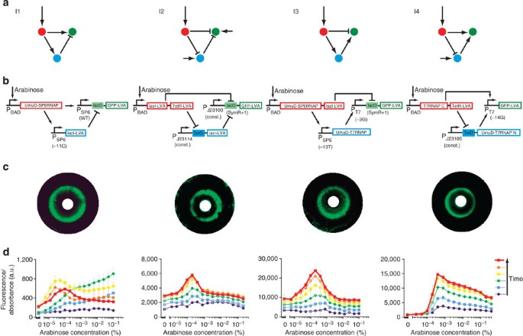Figure 4: The incoherent feedforward loop stripe-forming network family. (a) The four I-FFLs built (small arrow: constitutive promoter). (b) Implementations of the circuits in the network scaffold (Fig. 2). (c) Bacterial lawns display green fluorescent rings as a function of arabinose gradients from central paper disks (white)28,31. (d)E. colitransformed with each network display single fluorescent stripes in arabinose gradients as measured by fluorescence spectrometry (normalized by the absorbance). Time course for I1: 24-min intervals between each sample set, at 4–6 h of growth. For I2, I3 and I4: 12-min intervals, at 5–6 h of growth. Mean and s.d. from three biological replicates. Figure 4: The incoherent feedforward loop stripe-forming network family. ( a ) The four I-FFLs built (small arrow: constitutive promoter). ( b ) Implementations of the circuits in the network scaffold ( Fig. 2 ). ( c ) Bacterial lawns display green fluorescent rings as a function of arabinose gradients from central paper disks (white) [28] , [31] . ( d ) E. coli transformed with each network display single fluorescent stripes in arabinose gradients as measured by fluorescence spectrometry (normalized by the absorbance). Time course for I1: 24-min intervals between each sample set, at 4–6 h of growth. For I2, I3 and I4: 12-min intervals, at 5–6 h of growth. Mean and s.d. from three biological replicates. Full size image Quantitative mutant analysis and model fitting One of the challenges for synthetic biology is that real biological cells are vastly more complex than the simple circuits we wish to engineer. Therefore, our component parts may not work exactly as intended, or may interact with the cells’ native machinery causing unexpected dynamics [45] . It is therefore of central importance to show that an engineered circuit shows the desired behaviour using the expected mechanism and exclude any other mechanism. One advantage of our design space approach is that we know in advance that each of the four engineered circuits should be operating with a different dynamical mechanism [21] ( Fig. 1 ), which we can test ( Fig. 3b ). Thus, in Step 3, we confirmed each mechanism with two approaches: First, rather than just assaying the stripe pattern gene (from the GFP fluorescence; Fig. 4 ), we measured the activity of all three nodes of the network, using reverse transcription quantitative PCR of the messenger RNA (mRNA) levels at different concentrations of arabinose ( Fig. 5a ). Different mechanisms predict different spatial patterns of these intermediate genes (for example, in I1 the blue node shows a spatial gradient in the same orientation as the red node, while in I2 it is reversed; Fig. 1 ). Importantly, all results agreed with the predicted patterns ( Fig. 5a ). Second, we made a series of mutations to each core network, to alter quantitatively the effective strength of specific regulatory links. For each mutation, the expected impact on regulation was known from the literature ( Supplementary Fig. 7 ). In some cases, these mutations led to qualitative changes in the resulting GFP pattern (for example, the loss of the stripe in two of the mutations of I1, Fig. 5b ), while in others the GFP pattern was just quantitatively altered ( Fig. 5b ). 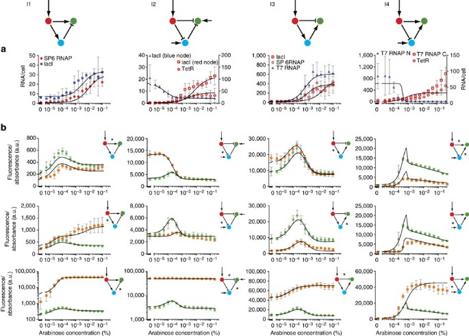Figure 5: Quantitative mutant analysis and model fitting. (a) Measured mRNA concentrations for all genes other than the stripe-forming gene at 6 h of growth. Mean and s.d. from three biological replicates. (b) Comparison of WT (green) and mutant (orange) network fluorescence at 6 h of growth. The interactions marked with an asterisk are modified in the mutant networks. The exact changes and conditions are listed inSupplementary Fig. 7. Mean and s.d. from three biological replicates. The black lines represent the model fitted simultaneously to the RNA data and fluorescence output of the WT and mutant networks for each design class. Figure 5: Quantitative mutant analysis and model fitting. ( a ) Measured mRNA concentrations for all genes other than the stripe-forming gene at 6 h of growth. Mean and s.d. from three biological replicates. ( b ) Comparison of WT (green) and mutant (orange) network fluorescence at 6 h of growth. The interactions marked with an asterisk are modified in the mutant networks. The exact changes and conditions are listed in Supplementary Fig. 7 . Mean and s.d. from three biological replicates. The black lines represent the model fitted simultaneously to the RNA data and fluorescence output of the WT and mutant networks for each design class. Full size image To confirm the mechanistic basis of each network class, we explored whether measurements from the individual nodes and all the mutated networks of each design class could be simultaneously fitted to the expected steady-state values of an ordinary differential equations computer model. The mathematical model uses the standard modelling approach [36] based on equilibrium binding of transcription factors to their sites on a promoter, where parameters refer to binding constants, Hill coefficients and transcription rates ( Supplementary Table 1 ), allowing thus for a comparison with existing values in the literature. While sharing a Hill-like mathematical expression, the regulation function used at Step 3 has more free parameters than the function from the complexity atlas exploration at Step 1. In Step 3, these free parameters acquire specific values through the fitting process, and thus characterize the specific biological conditions of the four constructs. This is in contrast to the exploratory, qualitative study of thousands of complex networks in Step 1, in which we fixed some of these parameters. Importantly however, the dynamical mechanism of stripe formation is conserved during this parameter reduction (see Supplementary Fig. 8 ). Employing the model, we asked whether it was possible to find a good fit in which only the mutated parameters are free to vary between the mutants, and the remaining regulatory parameters are required to be consistent across all networks. Good fits were obtained for all four network classes ( Fig. 5 , Supplementary Tables 2–6 ), indicating that they are indeed working according the four expected mechanisms. Moreover, the changes of the parameters predicted by fitting the mutant networks match the expected changes ( Supplementary Table 7 ). Finally, despite fitting each design class independently, a number of parameters are consistent across the study, suggesting that we have captured the universal aspects of these components ( Supplementary Table 8 ) and can use these parameters for the prediction of future networks. To our knowledge, such an extensive quantitative and multi-network verification of distinct mechanisms covering the complete design space has not been achieved before. The close match we achieved between theory and experiments gave us confidence in engineering further networks. For example, we built a variant of I2 with a positive feedback on the green node ( Supplementary Fig. 9 ). This network is located higher up in the complexity atlas than the minimal I2 network ( Fig. 1 ), and clearly has a different wiring design. However, it belongs to the same stalactite and is therefore expected to function with the same dynamical mechanism. Theoretical analysis of this particular design confirms this expectation and more importantly the synthetically constructed circuit also reveals the predicted dynamics over time and the spatial pattern of the intermediate genes ( Supplementary Fig. 9 ). Archetypal 2-node stripe-forming topology The success of building and modelling all four 3-node I-FFLs, led us to search for a deeper principle in the design space. Since all four designs contain both an activating and a repressing pathway between the morphogen sensor gene (red) and the stripe gene (green) we reasoned that it might be possible to achieve the stripe pattern with only 2 nodes. In this implementation, the first node would display both activator and repressor activities [46] which would act directly on the second node, but with different dynamics ( Fig. 6 ). We first used the computer model to confirm that such a simple network can indeed produce a stripe. This design represents the “archetype” of all I-FFL design classes—it can be envisioned as located just under the four 3-node networks in a complexity atlas and is thus a sub-stalactite ( Fig. 6a ). We therefore named this fundamental circuit ‘I-zero’ (I0). Most importantly, we were also successful in building this network synthetically ( Fig. 6 ) for the first time. We thus engineered the most elementary network capable of stripe formation, unifying the design space. 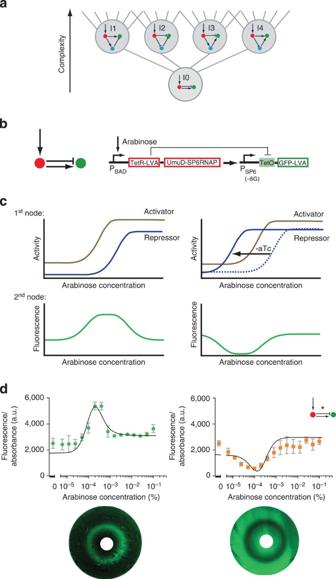Figure 6: Two-node archetypal stripe-forming network (I0). (a) I0 network complexity shown relative to the I-FFL stripe-forming family. (b) Circuit implementation in the network scaffold. (c) Schematic depictions of archetypal stripe (left) and anti-stripe (right) mechanisms. (d)E. colitransformed with the I0 network display a fluorescent stripe (left) or anti-stripe (right) in arabinose gradients, depending on the aTc concentration (0.125 μM for stripe, 0 μM for antistripe). Mean and s.d. from three biological replicates. The black lines represent the model fitted simultaneously to the RNA data and fluorescence output of the stripe, anti-stripe and a further variant at 5 h of growth (Supplementary Fig. 10). Corresponding bacterial lawns display a fluorescent ring or anti-ring as a function of arabinose gradients from central paper disks (white)28,31(bottom). Figure 6: Two-node archetypal stripe-forming network (I0). ( a ) I0 network complexity shown relative to the I-FFL stripe-forming family. ( b ) Circuit implementation in the network scaffold. ( c ) Schematic depictions of archetypal stripe (left) and anti-stripe (right) mechanisms. ( d ) E. coli transformed with the I0 network display a fluorescent stripe (left) or anti-stripe (right) in arabinose gradients, depending on the aTc concentration (0.125 μM for stripe, 0 μM for antistripe). Mean and s.d. from three biological replicates. The black lines represent the model fitted simultaneously to the RNA data and fluorescence output of the stripe, anti-stripe and a further variant at 5 h of growth ( Supplementary Fig. 10 ). Corresponding bacterial lawns display a fluorescent ring or anti-ring as a function of arabinose gradients from central paper disks (white) [28] , [31] (bottom). Full size image Modelling also predicted that the stripe output of the I0 network can be transformed into an ‘anti-stripe’. By strengthening the repressor activity, its dose–response curve shifts towards lower arabinose concentrations ( Fig. 6c ). In doing so, the effect of the repressor starts at a lower arabinose concentration than that of the activator. Given a moderate basal level of the activator, the resulting pattern is an anti-stripe. We were also able to confirm this prediction experimentally simply by lowering the concentrations of aTc (TetR regulator), thus increasing the effective concentration of the repressor ( Fig. 6d , Supplementary Fig. 7 , Supplementary Tables 2 and 7 ). Finally, we also demonstrated the power of our model to predict successfully the behaviour of further I0 mutants ( Supplementary Fig. 10 ). Building a network with non-native components performing a function of interest is a very strong evidence for the particular design rule [47] . In this study, we go beyond individual networks and explore both computationally and synthetically the whole design space of possible dynamical mechanisms for 3-node stripe-forming networks. For this purpose, we used a 3-step approach for the successful creation of synthetic circuits: first, we performed a theoretical screen for finding all design classes that produce the desired behaviour (stripe formation in a morphogen gradient). During this step we discovered four fundamentally different mechanisms for forming a stripe. We identified the minimal network for each mechanism and found that they correspond to the four known types of incoherent feedforward loops [35] , [48] (I1-I4). The Hill-like function model employed here differs from the connectionist-type of regulation function used in our previous analysis [21] . While the goal of our previous work was a qualitative exploration of stripe-forming networks, here we aimed for a quantitative comparison of the experimental data with a theoretical model. Therefore, the chosen model was a biologically- driven fine-grained one whose parameters have a measurable biological meaning (that is, transcription factor binding rate and transcription rates). Among the assumptions of the current model (see Supplementary Methods ), the introduction of constitutive promoters and AND-type signal integration produce inherent differences in the resultant complexity atlas when compared with the one from our previous work [21] . Next, we successfully built the four I-FFL networks synthetically. To this end, we developed a flexible network scaffold where the same components could be consistently used to build the different network topologies. The experience gained during building each network design (for example, the strengths of regulatory links) helped to build the subsequent ones. Consequently, each additional network took less time to tune the parameters for successful stripe formation, with the new scaffold enabling rapid testing of different parameter combinations. The establishment of the engineering criteria was also key to success, as they allowed straightforward identification and exclusion of stripes caused by metabolic load. The fundamental understanding of the mechanisms greatly simplified the engineering task, as we knew for each circuit with which dynamical mechanism it should be operating. The final step was to verify the distinct mechanisms by fitting all the experimental data to a mathematical model. In the last decade the synthetic biology has combined experiments and modelling aiming at an increasingly tighter relation between theory and data [49] . Often a qualitative theoretical model is fit to the experimental data [31] , [32] , [50] , without emphasizing the biological significance and values of the model’s parameters. However, there is also an extensive body of studies employing biologically derived theoretical models where the parameters have measurable, biological meaning such as binding and transcription rates [33] , [45] , [51] . In this work, we employed a model of the latter category and aimed for a quantitative agreement between theory and experiments. To achieve this goal we characterized the synthetic networks in unprecedented detail—by measuring the profiles of mRNA concentration for each gene and engineered derived variants for each design class and fitted all these data simultaneously to the mathematical model. As a result of this systematic and comprehensive approach the resulting fitted parameters were consistent across the study and to literature values. In other words, the modelling and quantitative fitting confirmed that we have a good match between theory and experiments across an entire design space (22 different networks representing various versions of the full family of incoherent feedforward motifs I1-I4 and I0) rather than just on a case-by-case basis. Another advantage of performing this study across the unified framework is that the system allowed us to explore mechanisms not yet discovered in nature. For instance, I3 and I4 forming a stripe had not been observed before in natural or synthetic transcriptional regulatory networks. The fundamental understanding of the mechanisms of the four stripe-forming design classes (I1-I4), led us to implement the archetype of I-FFLs stripe-forming networks (I0). This network is capable of reproducing the fundamental mechanism of stripe formation: staggered activator and repressor functions only allow net output gene expression at intermediate morphogen concentrations, resulting in a stripe. Shifting the dose–response curve of the repressor even allowed us to engineer an anti-stripe from the same minimal network, again demonstrating the close match between theory and experiments. We demonstrated here a framework for exploring and engineering within a unified network design space and showed that this can be more powerful than building networks one-by-one. An exhaustive analysis of the multiple ways of achieving the same phenotype allows more flexibility in a given synthetic biology project. Furthermore, understanding the mechanisms of the distinct design classes facilitates identifying the fundamental principles of a regulatory task. We have focused here on stripe formation from reading positional information in a morphogen concentration gradient. In the future, comprehensive computational and experimental exploration of genotype–phenotype maps has the potential to address other spatial and temporal patterns (for example, oscillations [52] ), as well as network properties [53] , [54] , [55] . Our approach thus provides a new and efficient recipe for synthetic biology. Network scaffold The three nodes of the network are contained in three compatible plasmids (pCOLA, pCDF, pET), each containing a multiple cloning sites ( Supplementary Fig. 11 ) for subcloning of the individual components ( Supplementary Fig. 12 ) and a set of transcriptional terminators. The plasmids contain different origins of replication (ori: ColA, CDF and pBR322) and antibiotic resistances (kanamycin, spectinomycin and ampicillin). The pCOLA plasmid constitutively expresses AraC and contains the P BAD promoter [56] . Therefore, the expression of genes cloned into this plasmid is induced by arabinose. The pET plasmid contains GFP (with a LVA degradation tag [57] ) for the fluorescent readout. Details of cloning ( Supplementary Methods ), plasmid maps ( Supplementary Fig. 13 ) and oligonucleotides sequences ( Supplementary Tables 9–13 ) are given in the Supplementary Information . The sequences of 16 plasmids used in this study have been submitted to GenBank with the accession codes KM229376-KM229391 ( Supplementary Fig. 13 ). E. coli strain A descendant of strain BW27783 (ref. 58 ) was used. In BW27783 the native araE promoter is replaced by a constitutive promoter. This results in a homogeneous cell population expressing genes under the control of the P BAD promoter, with a graded response to arabinose. In addition, in the strain used, lacI (ECK0342) was replaced by a chloramphenicol resistance gene (strain MK01 ref. 59 ) and tdk (ECK1233) was removed as previously described [60] . Fluorescence measurements Stripe experiments used ‘Stripe Medium’ (SM: 1 × Luria-Bertani (LB) medium plus 0.4% (w/v) glucose, 50 μg ml −1 ampicillin, 15 μg ml −1 kanamycin and 25 μg ml −1 spectinomycin). Spectinomycin was omitted for the I0 network, and 0.75 × LB was used for the I1 network. Three compatible plasmids were transformed simultaneously and the transformed bacteria were plated out on SM-agar plates. A single colony was picked for each biological replicate and grown overnight in 5 ml SM. The cultures were diluted to OD 600 0.0015 in SM (containing IPTG or aTc when indicated) and added to the wells of a 96-well plate (120 μl) together with arabinose (2.4 μl) at 16 different concentrations. The absorbance at 600 nm and green fluorescence (excitation: 485 nm, emission: 520 nm) were measured every 6 min in a Tecan Infinite M200 plate reader (37 °C, 220 s orbital (2 mm) shaking between readings) until the E. coli cells reached stationary phase (that is, the absorbance and fluorescence did no longer increase: 6 h for I1-I4, 5 h for I0). Both absorbance and fluorescence were background (SM only) corrected. The fluorescence was then normalized for the number of cells by dividing by the absorbance. RNA extraction Cells were grown in the Tecan plate reader as described in the section ‘Fluorescence measurements’ for 6 h (5 h for I0). 100 μl RNAprotect Bacteria Reagent (Qiagen) was added to 50 μl cells. The samples were mixed, incubated and centrifuged according to the manufacturer’s instructions. The cell pellets were stored at −80 °C until further processing. RNA was extracted using the Maxwell 16 LEV simplyRNA tissue kit (Promega). Briefly, the pellets were resuspended in 100 μl lysozyme (1 mg ml −1 in TE buffer, pH 8.0) and shaken for 5 min at room temperature. 100 μl of homogenization solution (including 1-thioglycerol) was added, followed by 200 μl of lysis buffer. A quantity of 2 ng of spike RNA and the cell lysates were transferred to the Maxwell cartridge and the remaining steps were performed by the Maxwell 16 instrument using the programme ‘simply RNA’. The RNA was eluted in 30 μl of water. The concentrations were determined by Nanodrop (ThermoScientific). The RNA was stored at −80 °C. RT–qPCR (reverse transcription quantitative PCR) A quantity of 700 ng of RNA was treated with Deoxyribonuclease I Amplification Grade (Invitrogen) according to the manufacturer’s instructions. A quantity of 8 μl of this reaction was directly used for reverse transcription using SuperScript III First-Strand Synthesis SuperMix for qRT–PCR (Invitrogen). The reaction was performed according to the manufacturer’s instructions, except for omitting digestion of the RNA with RNase H. The DNA was then quantified by qPCR (LightCycler 480 SYBR Green I Master, Roche) on a LightCycler 480 System (Roche). DNA amounts were determined with the help of a standard ladder of known quantities of the corresponding linearized plasmid. To obtain an estimate of mRNA copy numbers per cell, the cell lysates were spiked with a known amount (2 ng) of external RNA ( Supplementary Fig. 14 ). A recovery rate of the spike through the process of RNA extraction and RT–qPCR was calculated and applied to the other genes to obtain the initial amounts of mRNA copies per sample. To calculate the number of mRNA copies per cell, this number was divided by the number of cells present in a particular sample. Fluorescence measurements on agar plate For the detection of fluorescence from cells grown on an agar plate, we adapted previously described protocols [28] , [31] . Briefly, a single colony was picked and grown overnight in 5 ml SM. The OD 600 was measured and the culture was diluted to OD 0.15 in SM. 400 μl of the diluted culture were spread evenly over an SM-agar (1.5%, 20 ml) Petri dish (90 mm diameter). The SM-agar contained 15 μM IPTG for I2 and 0.2 μM aTc for the I0-stripe. The plates were incubated at 37 °C for 1 h. Subsequently, a dry 1 cm diameter autoclaved paper disc was placed at the centre of the plate and 15 μl of 5% (w/v) arabinose were injected onto the disc. The plates were incubated at 37 °C for another 6 h (5 h for the I0 anti-stripe network). Fluorescence images were acquired with a Typhoon Trio imager (GE Lifescience) using 488 nm laser excitation and 526 nm short pass filter detection; 200 μm resolution and agar top focusing (+3 mm). Grayscale images were converted to green using Image Quant TL software (GE Lifescience). The contrast was enhanced by using the curves function of Photoshop. Complexity atlas For the exploration of three-gene networks capable of forming a stripe, we employed a simulation code built in-house [21] . To adapt it to the current study, we used a Hill-like function model [36] for the gene regulation, allowing for both OR- and AND-type of signal integration at promoter level, as detailed in Supplementary Methods . We enumerated all possible three-gene networks with all interactions except self-inhibitions, and restricting only one gene to receiving the morphogen input. By using only the unique non-isometric topologies, there were 2,897 topologies to explore. When simulated with 100,000 random parameter sets each, 109 topologies showed a single-stripe pattern. The model and fitting procedure For the modelling and data fitting of the synthetic circuits we employed ROOT software (version 5.34— http://root.cern.ch ), a freely available customizable object-oriented C++ framework. Fitting in ROOT is based on the Minuit package that provides Maximum Likelihood Estimates through Local Optimization. We constructed a specific combined likelihood function associated to each of the five topologies, as described in Supplementary Methods . This function requires that parameters shared between mutants have identical values. In this way and from a given arabinose concentration, the function collectively fits the values of RNA/cell for each node of the circuit in all variants associated to the network (I0, I1, I2, I3, I4). The Hill-like function model [36] was used again. Accession codes : The sequences of 16 plasmids used in this study have been submitted to the GenBank nucleotide database under accession codes KM229376 to KM229391 . How to cite this article : Schaerli, Y. et al. A unified design space of synthetic stripe-forming networks. Nat. Commun. 5:4905 doi: 10.1038/ncomms5905 (2014).